Potential energy surfaces and reaction pathways for light-mediated self-organization of metal nanoparticle clusters Potential energy surfaces are the central concept in understanding the assembly of molecules; atoms form molecules via covalent bonds with structures defined by the stationary points of the surfaces. Similarly, dispersion interactions give Lennard-Jones potentials that describe atomic clusters and liquids. The formation of molecules and clusters can follow various pathways depending on the initial conditions and the potentials. Here we show that analogous mechanistic effects occur in light-mediated self-organization of metal nanoparticles; atoms are replaced by silver nanoparticles that are arranged by electrodynamic (that is, optical trapping and optical binding) interactions. We demonstrate this concept using simple Gaussian optical fields and the formation of stable clusters with various two-dimensional (2D) and three-dimensional (3D) geometries. The formation of specific clusters is ‘path-dependent’; the particle motions follow an electrodynamic potential energy surface. This work paves the way for rational design of photonic clusters with combinations of imposed beam shapes, gradients and optical binding interactions. Organization of metal nanoparticles (NPs) into ordered structures is one of the main pursuits of nanoscience, especially for applications in nanophotonics [1] , [2] , [3] . Many interesting optical properties, such as negative refraction and Fano resonance, are realized from the specific spatial arrangement of NPs and the resultant collective properties [4] , [5] , [6] . Top-down fabrication methods such as lithography are widely used to create ordered nanostructures [7] . However, these materials are often far from ideal with extensive defects and grain boundaries that alter and attenuate their properties due to the resulting strong dissipation [8] . By comparison, colloidal NPs can be (nearly) single crystals with a high degree of atomic and long range order [9] . These colloidal NPs would be better candidates to serve as building blocks [6] , yet spatial and temporal control of the positions of multiple colloidal NPs with nanometre precision is not easy to achieve due to random thermal forces (that is, Brownian motion) in solution. Optical tweezers offer one approach to control the position and orientation of single NPs [10] , [11] , [12] , [13] . The gradient force exerted by a tightly focused Gaussian beam can suppress Brownian motion and confine single Au or Ag NPs in solution [10] , [14] , [15] . Simultaneous control of multiple NPs is possible via holographic beam shaping using a spatial light modulator (SLM) [16] . Alternatively, (an array of) optical traps can be generated by localized surface plasmons in metallic nanostructures [17] or guided-resonance modes of photonic-crystal slabs [18] , leading to templated self-assembly of NPs. With an eye towards self-assembly in an applied field, sometimes termed self-organization, it is known that microparticles can spontaneously arrange themselves in a spatially extended optical field [19] , [20] , [21] , [22] by electrodynamic interactions termed ‘optical binding’ [19] . The spatial organization is an emergent property wherein the incident optical field is shaped by the light scattered from the particles thus creating a structured field that can, in turn, trap and localize more particles [23] , [24] , [25] , [26] . Recently, optical binding has been extended to Ag and Au NPs creating ordered arrays of metal NPs in a simple optical field [27] , [28] , [29] . These particles exhibit strong correlations in quasi-one-dimensional optical fields and act like rigid bodies. The strong electrodynamic (that is, optical binding) interactions suggest [30] an analogy to the concept of the Born-Oppenheimer potential energy surfaces (PESs) that govern molecular assembly, the formation of atomic clusters and liquids, and determine chemical reactivity [31] , [32] . Demonstrating the controlled self-organization of NP clusters in two and three dimensions with spatially shaped optical beams is a logical precursor to laser-induced molecular ‘assembly’ with controllable translational and orientational order [33] . Therefore, by analogy to the roles of PESs in molecular science, we demonstrate that control of the parameters of the incident optical field (shape, size, gradients, polarization) will give rise to different NP clusters by path-dependent assembly governed by the initial conditions (that is, positions) of the NPs accessing particular parts of the electrodynamic PES. Control by optical trapping and binding forces We begin by demonstrating that combinations of optical trapping and binding forces strongly and controllably influence the self-organization of Ag NPs. We used single Gaussian beam optical tweezers to trap Ag NPs with 100, 150 or 200 nm diameters near a coverslip surface ( Fig. 1a and Methods). As illustrated in Fig. 1b , we conducted optical trapping/optical binding studies of Ag NPs at a series of trapping planes (that is, planes of varying diameter in the Gaussian trapping beam) by altering the focal plane of the Gaussian beam with a virtual Fresnel lens created by an SLM ( Supplementary Note 1 ). 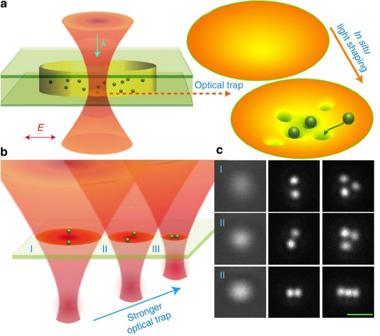Figure 1: Controlling NP arrangements by optical trapping and binding interactions. (a) Illustration of the sample cell and trapping beam, andin situlight shaping by Ag NPs trapped in the optical field. (b) Illustration of Ag NPs confined by focused Gaussian beams with different optical gradients near a transparent dielectric surface. The trapping planes I–III are 0.6 μm, 0.85 μm and 1.1 μm above the focal plane, respectively. (c) Optical images of the trapping planes (first column) and preferred arrangements of two and three 100 nm diameter Ag NPs (second and third columns) in the optical fields illustrated inb. Scale bar, 1 μm (seeSupplementary Movie 1). Figure 1c shows optical (darkfield microscopy) images of representative trapped NP clusters at different trapping planes obtained using the same NP size (100 nm). Different trapping forces were exerted on each Ag NP at these different planes ( Supplementary Fig. 1 ). For a weak optical trap (plane I), two Ag NPs tended to align perpendicular to the laser polarization (termed perpendicular and horizontal orientation in the images shown) as is also shown by the histograms in Supplementary Fig. 2 . This perpendicular dimer orientation is expected from optical binding [23] , [34] . However, when the trap was stronger (that is, NPs were confined closer to the focal plane), the preferred dimer orientation rotated (plane II) and could be made parallel to the polarization (plane III). Concomitantly, the equilibrium centre-to-centre separation of the NPs decreased, reflecting the stronger gradient forces from the optical beam. Therefore, for three NPs, the preferred arrangement was a triangle in a weak trap but a linear chain in a strong trap as shown in Fig. 1c . These results show that the forces that determine the structure of the Ag NP clusters in an optical field with gradients involve contributions from both optical binding and trapping (optical gradient) interactions. Figure 1: Controlling NP arrangements by optical trapping and binding interactions. ( a ) Illustration of the sample cell and trapping beam, and in situ light shaping by Ag NPs trapped in the optical field. ( b ) Illustration of Ag NPs confined by focused Gaussian beams with different optical gradients near a transparent dielectric surface. The trapping planes I–III are 0.6 μm, 0.85 μm and 1.1 μm above the focal plane, respectively. ( c ) Optical images of the trapping planes (first column) and preferred arrangements of two and three 100 nm diameter Ag NPs (second and third columns) in the optical fields illustrated in b . Scale bar, 1 μm (see Supplementary Movie 1 ). Full size image Light-mediated self-organization To explore the range of Ag NP cluster configurations that are obtained by self-organization via optical binding interactions, we chose an optical field with weak optical gradients (plane I in Fig. 1 ) to confine larger Ag NPs near the coverslip. 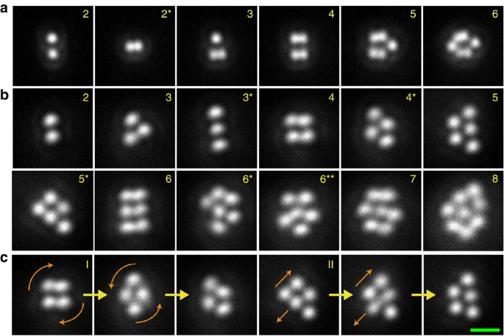Figure 2: Representative two-dimensional clusters formed by photonic self-organization. (a)~150 nm diameter NPs and (b) ~200 nm diameter NPs. (c) Structural transition between two configurations of photonic clusters with (I) four and (II) five NPs. The time interval between images is 0.01 s. Scale bar, 1 μm. The clusters were confined by a weak Gaussian optical field (plane I inFig. 1) near the coverslip, and the (linear) polarization direction is horizontal for all images (seeSupplementary Movies 2–7). Figure 2a,b summarize the equilibrium structures of clusters of up to eight Ag NPs with diameters of 150 and 200 nm. Some of the geometries, for example, the triangular cluster with one edge perpendicular to the polarization direction and the rectangular cluster of four NPs located on the vertices, were formerly only envisioned in theory [24] , [28] , [35] . Figure 2: Representative two-dimensional clusters formed by photonic self-organization. ( a ) ~ 150 nm diameter NPs and ( b ) ~200 nm diameter NPs. ( c ) Structural transition between two configurations of photonic clusters with (I) four and (II) five NPs. The time interval between images is 0.01 s. Scale bar, 1 μm. The clusters were confined by a weak Gaussian optical field (plane I in Fig. 1 ) near the coverslip, and the (linear) polarization direction is horizontal for all images (see Supplementary Movies 2–7 ). Full size image Most of the smaller clusters were very stable, behaving like a rigid body with little change of configuration. We determined the variance of the distribution of separations between optically bound dimers ( Supplementary Fig. 3 and Supplementary Note 2 ). The standard deviation decreased as the NP size increased—from 58 nm for 100 nm NPs to 7 nm for 150 nm Ag NPs to just 3 nm for 200 nm Ag NPs. In most cases, the clusters of larger Ag NPs (150 or 200 nm) did not fall apart for at least several minutes and they typically only changed if an additional particle was captured from solution. These rigid clusters include those shown in Fig. 2a-2 ( Supplementary Movies 2–6 ). Different stable configurations may exist for certain numbers of NPs, for example, different dimers of two 150 nm Ag NPs ( Fig. 2a-2 ) or different trimers of three 200 nm Ag NPs ( Fig. 2b-3 ) that would not interconvert. However, if a cluster had broken symmetry or similar structural isomers, it could switch between them. For example, the cluster in Fig. 2a-5 was observed to flip horizontally creating the mirror image structure and the left NP in Fig. 2b-6* could jump to the bottom site vacancy. Clusters with more NPs tended to transit (or even oscillate) between different configurations leading to structural fluctuations; for example, four 200 nm Ag NPs could oscillate between the two configurations shown in Fig. 2c-I ( Supplementary Movie 6 ) via a transitional structure (the diamond structure in the second panel that only exists in the transition), and five NPs could rapidly change their configuration via the sliding of NP pairs on the milliseconds time scale ( Fig. 2c-II ). There are also structural asymmetries associated with the direction of linear polarization of the trapping beam. For clusters of 150 nm Ag NPs, the inter-particle separation along the polarization axis or x axis (mean of the distributions of the inter-particle separations is <300 nm) is always smaller than that along the y axis (mean separations are 500–600 nm). For the 200 nm NPs, the difference is not so apparent. In addition to the intra-cluster properties, there are important attributes that we deduced for cluster growth. The self-organization has continuity, namely, the geometry of an N -particle cluster resembles that of an ( N –1)-particle cluster with an additional NP being added at a vacancy position. In addition, if a cluster of multiple NPs has only one equilibrium configuration, then it can be repeatedly built starting from a single NP (for example, Supplementary Movies 3,4 ). On the other hand, if two or more (stable) configurations are possible, the one formed would depend on the paths that the NPs enter the optical field ( Supplementary Movies 2,5,6 ). This kinetic trapping effect allows accessing structures that are not the global free energy minimum [36] . These observations suggest an Aufbau principle approach to calculating the equilibrium configurations. As described in Supplementary Figs 4–10 and Supplementary Notes 3,4 , we conducted electrodynamics simulations that reveal how the final structure of a cluster depends on the number and size of particles, as well as the gradient and polarization of the incident optical field. In the Methods section, we describe how the PESs are calculated from the optical forces. Path-dependent rules for assembly The most exciting observation is that the dynamics of self-organization of these optically bound clusters depends on the initial positions and hence paths the NPs take upon entering the optical field. We designed an experiment to demonstrate the path-dependent assembly for a particular set of NPs. We switched the optical trap between an annular optical field (that is, a ring trap) and a Gaussian trap so the same two NPs could be dissembled and reassembled many times ( Supplementary Movie 2 ). 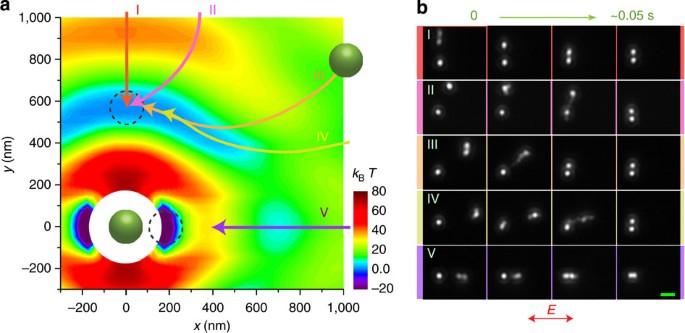Figure 3: Path-dependent self-organization of two Ag NPs. (a) Electrodynamic PES of two Ag NPs (150 nm diameter) and illustrated paths of the second particle entering the optical field. The units ofkBTassumeT=293 K. (b) The corresponding optical images of five trapping events where the second particle entered the optical field from different directions. Scale bar, 1 μm. Figure 3 shows five events where two 150 nm Ag NPs assembled into dimers along different paths resulting in different final structures; these paths are illustrated on a contour plot of the electrodynamic PES calculated for two 150 nm Ag NPs in a plane wave. In most cases (for example, events I–IV in Fig. 3b ), the two NPs formed a dimer at θ =90°. The only exception is if the second NP entered the trap very close to the x axis (for example, event V) then the NPs formed dimers at θ =0°. Note that θ =0° dimers had small inter-particle separations characteristic of the near-field regime; they were stabilized against aggregation to contact by the electrostatic repulsion of the polymer coating (that is, the dimer in Fig. 3b-V could still disassemble when the Gaussian field was removed). These paths and final structures are consistent with the PES shown in Fig. 3a ; specifically, whereas most pathways (starting from different orientational initial conditions) lead to the larger inter-particle separation along the y axis associated with optical binding, the thermal energy can only overcome the potential energy barrier and bring the second NP into near-field separation if its path is close to the x axis. (See Supplementary Note 5 on the thermal energies of laser-heated Ag NPs and Supplementary Note 3 on how the weak optical gradient modifies the energy barriers). Figure 3: Path-dependent self-organization of two Ag NPs. ( a ) Electrodynamic PES of two Ag NPs (150 nm diameter) and illustrated paths of the second particle entering the optical field. The units of k B T assume T =293 K. ( b ) The corresponding optical images of five trapping events where the second particle entered the optical field from different directions. Scale bar, 1 μm. Full size image The path-dependence of self-organization also applies in cases when there are more particles and they are of different sizes. For example, in the case of three 200 nm Ag NPs as shown in Fig. 4a,b , the PES shows two minima and the experiments also only exhibit two, corresponding to linear and near-equilateral triangular structures. The site the third particle finds depends on the initial position and path by which it enters the Gaussian field. This path-dependent rule also governs the self-organization of larger clusters. In Fig. 5a , we show the calculated PES for four Ag NPs (diameter 200 nm), which indicates several optical binding positions for the fourth particle. In the experiments, the fourth particle (for example, Fig. 4b.II-3 ) was indeed located near one of the predicted positions that is marked by a white asterisk in Fig. 5a . We did not observe clusters with the fourth particle located near the other two positions. The other two configurations lack centrosymmetry and thus are less stable in a Gaussian optical field where all the particles tend to move to the central area due to optical trapping forces (a central force). In the experiments the clusters actually shift their position in the trap such that their ‘centre of mass’ is centred in the cylindrically symmetric trap potential, so centrosymmetric structures are favoured. Trapezoidal (diamond-like) and square structures are shown in Fig. 2 and the relatively low barriers to structural conversion that are implied in Fig. 5 are also manifest in the experimental data. Together, the results of Figs 3 , 4 , 5 indicate that the most probable locations where an additional Ag NP joins an existing cluster can be predicted from the electrodynamic PES calculated for the appropriate imposed beam shape and number of particles. 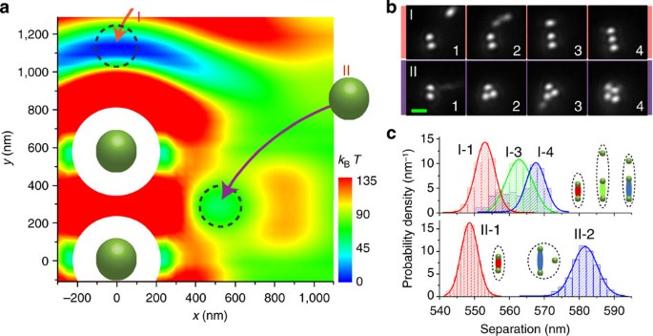Figure 4: Path-dependent self-organization of three Ag NPs. (a) Electrodynamic PES of the third Ag particle joining an optically bound dimer (200 nm diameter) in an optical field, and illustrated pathways of the third Ag NP. (b) The corresponding images of two trapping events where the third particle entered the optical field from different directions. The images II-3 and II-4 further show the addition of a fourth NP. The relative time points of the images in I are 0 s, 0.01 s, 0.02 s and 1.82 s; and that in II are 0 s, 0.01 s, 0.66 s and 0.67 s, respectively. Scale bar, 1 μm. (c) Histograms of the centre-to-centre distances between the first two NPs before and after the third one joined, corresponding to the two cases shown inb. Parameters of the corresponding Gaussian fits of the histograms are shown inSupplementary Table 1. Figure 4: Path-dependent self-organization of three Ag NPs. ( a ) Electrodynamic PES of the third Ag particle joining an optically bound dimer (200 nm diameter) in an optical field, and illustrated pathways of the third Ag NP. ( b ) The corresponding images of two trapping events where the third particle entered the optical field from different directions. The images II-3 and II-4 further show the addition of a fourth NP. The relative time points of the images in I are 0 s, 0.01 s, 0.02 s and 1.82 s; and that in II are 0 s, 0.01 s, 0.66 s and 0.67 s, respectively. Scale bar, 1 μm. ( c ) Histograms of the centre-to-centre distances between the first two NPs before and after the third one joined, corresponding to the two cases shown in b . Parameters of the corresponding Gaussian fits of the histograms are shown in Supplementary Table 1 . 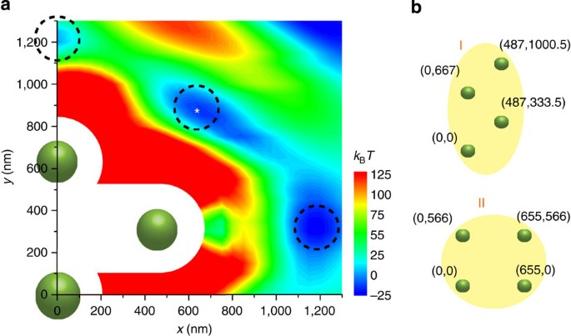Figure 5: Self-organization of four Ag NPs. (a) Electrodynamic PES of the fourth Ag particle joining an optically bound trimer (200 nm diameter) in an optical field. (b) Equilibrium arrangements of four Ag NPs in the optical field; (x, y) coordinates are indicated. Full size image Figure 5: Self-organization of four Ag NPs. ( a ) Electrodynamic PES of the fourth Ag particle joining an optically bound trimer (200 nm diameter) in an optical field. ( b ) Equilibrium arrangements of four Ag NPs in the optical field; ( x, y ) coordinates are indicated. Full size image In fact, the predicted geometry with an asterisk ( Fig. 5a ) is slightly different from the stable and symmetric structure observed in the experiments. This reveals an important aspect of the self-organization of the Ag NPs; that is, the scattered light from the new NP will also modify the overall optical field, and thus disturbs the equilibrium configuration of the pre-existing cluster of N–1 particles. This effect is demonstrated in Fig. 4c , where the addition of a third particle always increases the separation of the two NPs in an existing dimer. As the forces on the pre-existing NP nucleus will no longer be zero, the geometry of the calculated final cluster was determined by iterative optimization using an algorithm described in Supplementary Note 4 to optimize the arrangement by simulation. The basic idea is to move each NP in the direction of optical force exerted on it until all the NPs converge to equilibrium. The obtained equilibrium arrangements of four Ag NPs in a plane wave are shown in Fig. 5b , which resemble the two configurations observed in the experiments. Of course, the PES for the dynamics of assembly and organization needs to be adiabatically modified in an analogous manner but implementing this is beyond the scope of the present study. 3D photonic clusters Although the results have thus far focused on the formation of 2D photonic clusters, it is important to understand that our methodology also generates 3D optically bound photonic clusters. Generally 2D photonic clusters are more stable than 3D clusters due to the strong optical scattering forces that tend to push the NPs close to the coverslip surface. However, if the size of a 2D cluster consisting of multiple NPs becomes comparable with the size of the optical trapping field, then the peripheral NPs may jump back to the central area of the beam. However, as the optimal locations (at the focal plane near the glass surface) are occupied, the fluctuating NP moves to a different z -plane leading to a 3D photonic cluster whose structure is defined by the mutual interactions of all the NPs. Identifying 3D clusters is not easy though because of the projection of volume information to 2D detectors. However, if we record a sequence of images and thus know the particle number in a certain cluster, then it is possible to determine if the cluster has a 2D or 3D structure and estimate the 3D structure. In Fig. 6 (also see Supplementary Movie 8 ), we show the formation of three different Ag NP clusters that at some point become 3D clusters with the structures illustrated on the right side. In each case, a 2D cluster forms at the beginning, and then an NP jumps on the top of the 2D cluster and becomes brighter, forming a 3D structure. The increased brightness is consistent with our earlier work on co-trapping of semiconductor quantum dots in electrodynamic hot spots created by interference of scattering from a rigid chain of NPs and the incident optical trapping beam [29] . Note that in the cases of Fig. 6b,c , by just considering the particle size and cluster geometry, there is a possibility that the NP may locate in the empty 2D space between the three or four NPs (as seen in the x-y view). However, this is not allowed by the strong electrostatic and electrodynamic repulsions between the NPs. 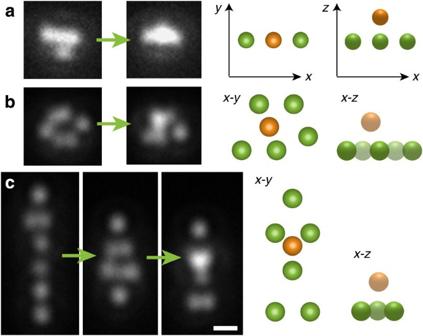Figure 6: Three-dimensional (3D) clusters formed by photonic self-organization. Optical images that show the formation of 3D photonic clusters (in the rightmost panels) and the corresponding illustrations of the 3D structures. The green and orange colours indicate Ag NPs at differentzplanes. (a) Four 100 nm diameter Ag NPs confined by a focused Gaussian beam (plane III inFig. 1). (b) Six 150 nm diameter Ag NPs confined by a focused Gaussian beam (plane I inFig. 1). (c) Seven 150 nm diameter Ag NPs confined by an optical line trap. The long axis of the line trap is along they-direction. Scale bar, 500 nm. Note that we do not have precise information about thezaxis positions so the illustrated structures are best estimates judging from changes in the focusing and particle brightness29. Figure 6: Three-dimensional (3D) clusters formed by photonic self-organization. Optical images that show the formation of 3D photonic clusters (in the rightmost panels) and the corresponding illustrations of the 3D structures. The green and orange colours indicate Ag NPs at different z planes. ( a ) Four 100 nm diameter Ag NPs confined by a focused Gaussian beam (plane III in Fig. 1 ). ( b ) Six 150 nm diameter Ag NPs confined by a focused Gaussian beam (plane I in Fig. 1 ). ( c ) Seven 150 nm diameter Ag NPs confined by an optical line trap. The long axis of the line trap is along the y -direction. Scale bar, 500 nm. Note that we do not have precise information about the z axis positions so the illustrated structures are best estimates judging from changes in the focusing and particle brightness [29] . Full size image Our optical trapping experiments and electrodynamic simulations reveal the multi-facetted role of optical gradients that strongly affect the self-organization. There is an active tension between the overall centrosymmetric optical gradient used here and the more nuanced optical binding interactions. Previous theoretical work generally ignored the role of optical gradients and only considered optical binding in plane waves [23] , [28] , [30] , [35] , but in practice, optical gradients are necessary to confine NPs to form clusters (for example, to counteract diffusion). The geometries of the photonically organized clusters depend on the mutual contributions of optical trapping and binding forces, the optical trap shape, the polarization of the light (and torque it can exert), the electrostatic force, as well as the paths that the particles take on entering the optical field. Thus, the self-organization is a complex dynamic process. In fact, although there may be many cluster geometries satisfying the electrodynamic equilibrium for a certain number of NPs [28] , [35] , not all the geometries are experimentally accessible. Still, the equilibrium geometries and pathways for assembly measured in experiment agree with what is expected from electrodynamic simulations and, in particular, the electrodynamic PESs constructed from our simulations. These results can help in interpreting different lattice configurations of optically bound particles in previous reports [21] , [22] , and serve as a guideline for future research. Our observation of unusual lattices, such as meso-scale rectangular clusters that are otherwise inaccessible via chemical approaches, suggests that the photonic self-organization of metal NPs will provide new opportunities to build artificial nanostructures tailored for particular applications. The field enhancement due to mutual scattering and interference from the 2D and 3D clusters can generate hot spots away from the NP surface [29] , and different arrangements of NPs and their spacing would lead to enhancement of different wavelengths at a certain position. This opens up new practical avenues in sensing that do not require analyte binding to NPs but rather that will allow flow through dynamically reconfigurable arrays. This would represent a totally different scenario from the current sensor and spectroscopy enhancements (for example, Raman, SERS) that are all near-field and essentially require molecules to be stuck or localized on the NPs. Furthermore, we are interested in applying the photonic clusters in quantum optics research. For example, could the photonic clusters modulate the radiative rate of excitons by controlling the coupling of quantum dots co-trapped by the metallic clusters? One exciting prospect of 3D structures is to create photonic bandgap materials as compared with stopbands that are possible in 2D [37] , [38] . Such structures could be the basis for Purcell enhancement and diminution. Finally, our experiments and electrodynamic simulations provide a new way of viewing and possibly even directly simulating NP dynamics in applied fields as arising from classical or Langevin dynamics. For these reasons, this paper represents a first step in the rational design of photonic clusters with nanometre scale precision in optical fields with appropriate optical beam shapes and gradients. Particles The Ag NPs were purchased from nanoComposix, Inc. The reported diameters for the 100 nm Ag NPs are 99±6 nm and are coated by polyvinylpyrrolidone with a zeta potential of −37.4 mV. The diameters for the 150 nm Ag NPs are 151±13 nm and are coated by citrate with a zeta potential of −56.2 mV. The diameters for the 200 nm Ag NPs are 203±24 nm and are coated by polyvinylpyrrolidone with a zeta potential of −34.7 mV. The colloidal solutions were diluted with deionized water and filled into a sample cell consisting of a spacer forming a chamber between two coverslips. The coverslips were UV/Ozone treated to make their surface negatively charged so that the repulsive electrostatic force prevented the NPs from being stuck on the surface. Optical tweezers The experiments were conducted with an optical tweezers apparatus [28] . An 800-nm Gaussian beam generated by a Ti:sapphire laser was initially focused onto the coverslip by a × 60 water-immersion objective (Olympus UPLSAPO, NA=1.2). Note that in the actually experiment, the incident beam was upward and the particles were in a plane defined by the top (upper) coverslip of the sample cell. The illustrations in Fig. 1 were inverted for better visualization. The laser power before the objective was measured to be ~60 mW. To select different optical planes for optical trapping, we used a SLM (Hamamatsu Photonics X10468 Series) to apply Fresnel lens phase marks with different focal lengths to the laser beam. We also produced a ring trap to dissemble the Ag NP clusters from those formed in the Gaussian beam, but still confine the NPs in the work plane, and reassembled them by switching back to the Gaussian beam. The NPs were visualized by darkfield microscopy with a high NA darkfield condenser (Olympus, U-DCW, NA=1.4), and recorded using a scientific CMOS camera (Andor Neo) with frame rate of 100 fps. Trajectories of the NPs were extracted by fitting the image of each NP with a 2D Gaussian function using commercial software (DiaTrack). Electrodynamics simulations Optical forces on Ag NPs in optical fields were calculated using Lumerical ‘FDTD Solutions’ software. The Ag spheres (refractive index 0.04+ i 5.57) are immersed in water (refractive index 1.33) and illuminated by a linearly polarized plane wave or a Gaussian beam with λ =800 nm (vacuum). When a Gaussian beam is used for a two-particle system, the centre of the beam is always set at the midpoint between the two NPs as this corresponds to the experimental observations. To obtain the correct force magnitudes, the light intensity is assumed to be 23.6 mW μm −2 , corresponding to that of the defocused Gaussian beam used in our experiments ( Supplementary Note 5 ). (Of course the electrodynamics results simply scale linearly with intensity and so any value could be used in the actual numerical calculations.) The Ag spheres are always in the x-y plane and the light propagates in the z direction with polarization along the x axis. A non-uniform mesh with maximum grid size of 5 nm was used. When calculating the force maps, we start from two NPs and fix the position of one while scanning the position of the other one in the x-y plane. The optical forces are calculated by integrating the Maxwell stress tensor over a surface surrounding the NP [12] . Once the optical binding position of the second NP is known, we can place the NP there and calculate the force map for the third one. Note that for multiple NPs, the binding positions need to be optimized as described in the Supplementary Note 4 . PESs are calculated by integrating the forces along defined paths via the formula: where s parameterizes any path in ( x , y ) such that s =0 corresponds to a reference position P 0 =( x 0 , y 0 ) and s =1 corresponds to arbitrary point P '=( x ′, y ′). For example, the potential at an arbitrary point of ( x ′, y ′) in Fig. 3a is obtained by setting x 0 =1,000 nm and y 0 =1,000 nm and employing a path that corresponds to integrating in x from x = x 0 to x ′ with y fixed at y 0 , and then integrating in y from y = y 0 to y ′ with x fixed at x 0 . For visualization, the resultant PES is finally shifted by setting the potential of the stationary point on the y axis as zero. How to cite this article: Yan, Z. et al. Potential energy surfaces and reaction pathways for light-mediated self-organization of metal nanoparticle clusters. Nat. Commun. 5:3751 doi: 10.1038/ncomms4751 (2014).